A multi-omic map of the lipid-producing yeastRhodosporidium toruloides Triacylglycerols are among the most attractive alternative raw materials for biofuel development. Current oil plant-based technologies are limited in terms of triacylglycerol production capacity and rate. These limitations may be circumvented by biotransformation of carbohydrates into lipids; however, our understanding of microbial oleaginicity remains limited. Here we present the results of a multi-omic analysis of Rhodosporidium toruloides , a robust triacylglycerol-producing fungus. The assembly of genome and transcriptome sequencing data reveals a genome of 20.2 Mb containing 8,171 protein-coding genes, the majority of which have multiple introns. Genes including a novel fatty acid synthase are predicted to participate in metabolic pathways absent in non-oleaginous yeasts. Transcriptomic and proteomic data suggest that lipid accumulation under nitrogen-limited conditions correlates with the induction of lipogenesis, nitrogenous compound recycling, macromolecule metabolism and autophagy. The multi-omic map of R. toruloides therefore provides a valuable resource for efforts to rationally engineer lipid-production pathways. Triacylglycerols (TAGs) are neutral lipids that are naturally produced via fatty acid biosynthetic pathways. TAGs are used as foods, animal feeds and feedstocks for chemical syntheses [1] . Recently, derivatives of TAGs, such as long-chain fatty acid methyl esters [2] and alkanes [3] , have been explored as drop-in biofuels. However, traditional technologies that are based on oil crops and plants are limited in terms of their production capacity and rate. The harnessing of microbial fatty acid biosynthetic machineries may circumvent those limitations [4] , [5] . Some oleaginous species are exceptionally robust in converting carbohydrates into lipids, such as TAGs [6] . Yeast species of the anamorphic genus Rhodotorula have often been used for transformation of renewable resources into microbial oils [7] , [8] , [9] . Rhodosporidium toruloides (formerly known as Rhodotorula glutinis or Rhodotorula gracilis ), which is a non-pathogenic, pink-coloured basidiomycetous fungus, can accumulate lipids to more than 70% of its dry cell weight [6] , [10] . This 'red' yeast is also a good producer of carotenoids [11] and biotechnologically important enzymes, such as cephalosporin esterase [12] and epoxide hydrolase [13] . More importantly, R. toruloides has excellent tolerance of inhibitory compounds that are found in biomass hydrolysates [14] . Thus, R. toruloides is a unique yeast strain of great biotechnological potential. Although a copious literature presenting the results of lipid production by oleaginous species exists [6] , [15] , the understanding of the molecular basis of microbial oleaginicity and the sparse capacity for rational strain engineering is limited, largely because genetic backgrounds of naturally oleaginous species remain poorly documented. Next-generation DNA sequencing technologies enable rapid genome decoding, high-throughput transcriptome sequencing (RNA-seq) [16] and gene expression profiling (3′-Tag sequencing) [17] . Furthermore, advances in mass spectrometry-based proteomic analysis allow for the identification of thousands of proteins in a single experiment. The mystery of microbial oleaginicity may be unearthed using a natural lipid producer and an in-depth study that integrates the above-mentioned state-of-the-art technologies [18] , [19] , [20] . Here we present the results of genomic sequencing of R. toruloides , and differential transcriptomic and proteomic analyses of samples that were prepared under various culture conditions. We show that lipid accumulation under nitrogen-limited conditions is tightly connected with cellular processes that are related to lipogenesis, macromolecule metabolism and autophagy. We also find novel genes and pathways (such as fatty acid synthesis and lipid storage) that are committed to oleaginicity. Much information is consistent at different omic levels, and such multi-omic data significantly enriches our understanding of the molecular basis of lipid accumulation. This should facilitate the engineering of a natural lipid producers and other microorganisms for improved efficiency, robustness and economics of the microbial production of fatty acid derivatives. Genomic and transcriptomic sequencing and annotation The genome of the haploidic strain R. toruloides NP11 was sequenced using the Illumina sequencer platform ( Supplementary Table S1) , and the de novo sequence assembly resulted in a 20.2-Mb genome with an average coverage of 96× ( Supplementary Fig. S1 ) and 94 scaffolds (>1 kb, L50=575 kb, Supplementary Table S2 ). After PCR-based gap closure, the genome was narrowed down to 34 scaffolds, which included one ribosomal DNA unit sequence ( Supplementary Fig. S2 and Supplementary Table S2 ). The genome was organized into 16 chromosomes that ranged from 650 to 1900 kb ( Supplementary Fig. S3 and Supplementary Methods ). To validate the completeness of the genome assembly and to define the transcriptional landscape of R toruloides , the transcriptome was sequenced using RNA-seq, which generated 6.7 M paired-end reads ( Supplementary Table S1 ). It was found that 79% of the sequenced complementary DNA (cDNA) fragments and 98.6% of the assembled expressed sequence tags could be mapped to the genome. Moreover, except for KOG1185 and KOG1394, which are absent in basidiomycetous fungi, 246 of the 248 core eukaryotic genes [21] were found. These results indicated that the assembled genome encompassed a very high percentage of the gene space. The repetitive sequences constituted 1.66% of the current assembly ( Supplementary Table S3) , and RNA-seq alignment combined with de novo gene prediction, homology search and manual curation resulted in the prediction of 8,171 protein-coding genes ( Supplementary Fig. S4 and Supplementary Table S4 ). The gene-coding regions were considerably dense with an average of 2.6 kb per gene. In addition, similar to other basidiomycetous fungi, split genes, which have short and multiple introns, were predominant, and 7,938 genes were found to have at least one intron. Moreover, most genes with 5′- and 3′-untranslated regions were annotated with the assistance of RNA-seq ( Supplementary Table S4 ). It was found that 90% of the gene models had more than 30% of their length covered by RNA-seq reads, which were mapped to the annotated open-reading frames using the Bowtie software [22] , and 38% of the annotated proteins had at least one unique peptide that was present at the proteomic level ( Supplementary Table S5 ). RNA-seq data indicated that 1,371 genes encoded two or more transcript isoforms, suggesting that the transcriptome was more complex than that of the static genomic data set ( Supplementary Fig. S5 ). For the functional annotation, 79% of the R. toruloides proteins had homologous proteins or conserved domains of known proteins ( Supplementary Table S5 ). Approximately 60% of proteins were annotated with Gene Ontology (GO) terms, and 32% of proteins were found with KEGG (Kyoto Encyclopedia of Genes and Genomes) orthology numbers. On the basis of these annotations, we reconstructed the central and lipid metabolism of this organism ( Fig. 1 ). In comparison with Saccharomyces cerevisiae , R. toruloides contains ATP:citrate lyase (ACL), and the mitochondrial β-oxidation (MBO) and carotenoid biosynthetic pathways. Although cytoplasmic acetyl-CoA synthase can produce acetyl-CoA from acetate, in oleaginous fungi and higher eukaryotes, acetyl-CoA, which results from the cleavage of citrate by ACL, is a major source for lipid synthesis [23] . Unlike β-oxidation in peroxisomes, the MBO pathway recovers more energy through the degradation of fatty acids by using the flavin adenine dinucleotide (FAD) cofactor, which couples with the respiratory chain to produce ATP. Moreover, MBO-associated enzymes are required to metabolize branched-chain amino acids to produce acetyl-CoA [24] , [25] . Thus, MBO may provide alternative acetyl-CoA and energy sources for fatty acid synthesis by degrading amino acids and membrane lipids (vide infra). Two genes that code putative carotenoid synthesis-related enzymes, phytoene synthase ( PSY1 ) and phytoene dehydrogenase ( CRTI ), were identified, revealing the genetic basis for the formation of the pink-coloured pigments by this organism ( Supplementary Fig. S6 a ). 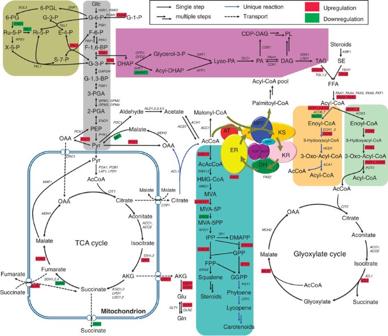Figure 1: Reconstruction of central and lipid metabolism pathways ofR. toruloides. The metabolic network that was reconstructed from the KEGG pathway and SGD annotation (http://www.yeastgenome.org/) included glycolysis (grey), the pentose phosphate pathway (olive), the TCA cycle, fatty acidde novosynthesis, isoprenoid biosynthesis (blue), triacylglycerol and phospholipid biosynthesis (purple) and lipolysis, β-oxidation in mitochondria (orange) or peroxisomes (pale green) and the glyoxylate cycle. Metabolic reactions that were present inR. toruloidesbut absent inS. cerevisiaeare indicated with blue arrows, and upregulation and downregulation of genes in response to nitrogen depletion are highlighted in red and green, respectively. Abbreviations for the components of the fatty acid synthase system are ACP, acyl carrier protein; AT, acyltransferase; DH, dehydratase; ER, enoyl reductase; KR, ketoacyl reductase; KS, ketoacyl synthase; MPT, malonyl/palmitoyl transferase; PPT, phosphopantetheine transferase. More abbreviations, gene symbols, annotations and expression abundance data are included inSupplementary Tables S8 and S9. Figure 1: Reconstruction of central and lipid metabolism pathways of R. toruloides . The metabolic network that was reconstructed from the KEGG pathway and SGD annotation ( http://www.yeastgenome.org/ ) included glycolysis (grey), the pentose phosphate pathway (olive), the TCA cycle, fatty acid de novo synthesis, isoprenoid biosynthesis (blue), triacylglycerol and phospholipid biosynthesis (purple) and lipolysis, β-oxidation in mitochondria (orange) or peroxisomes (pale green) and the glyoxylate cycle. Metabolic reactions that were present in R. toruloides but absent in S. cerevisiae are indicated with blue arrows, and upregulation and downregulation of genes in response to nitrogen depletion are highlighted in red and green, respectively. Abbreviations for the components of the fatty acid synthase system are ACP, acyl carrier protein; AT, acyltransferase; DH, dehydratase; ER, enoyl reductase; KR, ketoacyl reductase; KS, ketoacyl synthase; MPT, malonyl/palmitoyl transferase; PPT, phosphopantetheine transferase. More abbreviations, gene symbols, annotations and expression abundance data are included in Supplementary Tables S8 and S9 . Full size image A novel fatty acid synthase (FAS) system was found in R. toruloides ( Fig. 2 ). FASs are typically classified into two variants, the dissociated type II system and the integrated type I multi-enzyme. In fungi, FASs are usually composed of eight distinct domains and organized into two subunits or one polypeptide [26] . Although split FASs are common in fungi, FAS in R. toruloides is split into a novel form that consists of two subunits: the β-subunit (Fas1), which contains acyltransferase and enoyl reductase domains, and the α-subunit (Fas2), which includes all other domains ( Fig. 2a ). Two acyl carrier protein (ACP) domains of 76% sequence identity are present in Fas2, and these two ACPs share high similarity with ACPs from other species ( Supplementary Figure S7 ). Unique peptides from different ACPs were also found by LC-MS/MS (liquid chromatography–mass spectrometry) during proteomic analysis ( Fig. 2b ; Supplementary Fig. S8 ), which unambiguously indicated the expression of the FAS with two ACPs. As ACP has a key role in iterative substrate shuttling in the chain-elongation process, the presence of tandem ACPs may improve the efficacy of fatty acid biosynthesis by providing a higher intermediate concentration in the reaction chamber of FAS [27] . 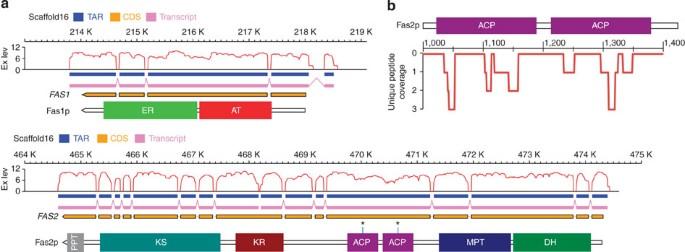Figure 2:R. toruloidesfatty acid synthase system. (a) Schematic representation of the transcriptional map and domain architecture of FAS. TheFAS1andFAS2genes localized to the same scaffold and were separated by approximately 250 kb, and the entire transcripts were reconstructed from RNA-seq data. TAR, transcription active region; Transcript, reconstructed transcript; CDS, coding sequence; Ex lev, expression level, log2(RNA-seq reads coverage); AT, acyltransferase; ER, enoyl reductase; DH, dehydratase; MPT, malonyl/palmitoyl transferase; ACP, acyl carrier protein; KR, ketoacyl reductase; KS, ketoacyl synthase; PPT, phosphopantetheinyl transferase. Asterisks represent the conserved serine residues for 4′-phosphopantetheine attachment. (b) Unique peptide coverage that was identified by LC-MS/MS. Figure 2: R. toruloides fatty acid synthase system. ( a ) Schematic representation of the transcriptional map and domain architecture of FAS. The FAS1 and FAS2 genes localized to the same scaffold and were separated by approximately 250 kb, and the entire transcripts were reconstructed from RNA-seq data. TAR, transcription active region; Transcript, reconstructed transcript; CDS, coding sequence; Ex lev, expression level, log 2 (RNA-seq reads coverage); AT, acyltransferase; ER, enoyl reductase; DH, dehydratase; MPT, malonyl/palmitoyl transferase; ACP, acyl carrier protein; KR, ketoacyl reductase; KS, ketoacyl synthase; PPT, phosphopantetheinyl transferase. Asterisks represent the conserved serine residues for 4′-phosphopantetheine attachment. ( b ) Unique peptide coverage that was identified by LC-MS/MS. Full size image Transcriptomic analysis Early biochemical studies demonstrated that nitrogen limitation was a major regulator for initiating lipid overproduction ( Supplementary Fig. S6 d,f,g ) [6] , [10] . In oleaginous fungi, mitochondrial NAD + -dependent isocitrate dehydrogenase (IDH) is dependent on adenosine monophosphate (AMP), and under nitrogen limitation conditions the cellular AMP level is lowered because of AMP deaminase activity, which leads to an impaired activity of IDH. Consequently, mitochondrial citrate accumulates and permeates out from the mitochondria to the cytosol where it serves as a substrate for ACL to form acetyl-CoA for fatty acid biosynthesis. In addition, cytosolic NADP + -dependent malic enzyme (ME) is considered as the key enzyme that supplements nicotinamide adenine dinucleotide phosphate (NADPH) for de novo lipogenesis. In addition to lipid accumulation, nitrogen limitation is expected to mediate a more global response, such as the release of nitrogen catabolite repression (NCR) [28] and the induction of autophagy by the target of rapamycin (TOR) signalling cascades [29] , [30] . We grew chemostat cultures of R. toruloides to examine the influence of nitrogen starvation on this organism ( Table 1 ). In a minimal medium with abundant ammonium (MM), cells accumulated lipids to 22.8%, and the residual ammonium concentration was 47±1 mM. In minimal medium with trivial amounts of ammonium (MM-N), the cellular lipid content was 33.3%. Furthermore, the oil yield, which was based on consumed sugar ( Y SP ), in the MM-N medium was 3.6-fold higher than that in the MM medium. These results clearly indicated that nitrogen limitation promoted lipid accumulation and that the metabolic flux was repartitioned for lipid biosynthesis. Table 1 Parameters and results of R. toruloides cultures. Full size table The 3′-tag digital gene expression (DGE) profiling experiment produced more than three million tags from each RNA sample that was prepared from cells cultured in the MM or MM-N media ( Supplementary Table S1 ). Of those tags, 78% from the MM sample and 63% from the MM-N sample mapped to annotated transcripts, and 89% from the MM sample and 74% from the MM-N sample mapped to the genome ( Supplementary Table S6 ). In addition, 5.7% of those tags mapped to antisense transcripts of predicted genes, which led to the observation that 74% of the total genes exhibited antisense transcription ( Supplementary Table S6 ). These data indicated that antisense transcription is widespread in R. toruloides . Approximately 12% of the reads that uniquely mapped to sense transcripts were not aligned to the 3′-most Nla III site ( Supplementary Figure S9 ), which suggested that transcription at the 3′-end was heterogeneous. For transcript quantification, the tags that mapped to sense sequences were counted and compared. Of the 7,045 genes that were expressed in these two samples ( Supplementary Table S6) , 1,177 and 853 genes were significantly upregulated and downregulated, respectively ( Fig. 3a ). It was obvious that nitrogen limitation influenced a variety of cellular processes such as metabolism, localization and transportation ( Fig. 3b ). NCR-related genes were induced ( Fig. 3c ), and MEP2 , which is the orthologue of the S. cerevisiae high-affinity ammonia transporter, was upregulated tenfold. In addition, three genes that coded amino acid permeases ( RHTO_00398 , RHTO_00931 and RHTO_01882 ) were upregulated. The central nitrogen metabolism machinery, which is composed of glutamate dehydrogenase (GDH), glutamine synthase (GLN) and glutamate synthase (GOGAT/GLT), is the hub of cellular nitrogen utilization, and it was discovered that the transcription of GDH1 , GDH2 and GLN1 were upregulated under nitrogen-limited conditions. It was also found that the expression of genes involved in urate and urea degradation was upregulated, whereas the expression of genes related to the utilization of other poor nitrogen sources was not significantly altered ( Supplementary Table S7 ). Furthermore, genes coding proteases ( PRB1 and PEP4 ) and amino acid permeases ( RHTO_05155 and RHTO_02128 ) that are linked to vacuolar protein degradation were induced. As Pep4 activates other vacuolar hydrolases, this elevated expression level would enhance the degradation of macromolecules and organelles. Indeed, autophagy-related genes ( ATG1 , ATG2 , ATG20 and ATG8 ) and vacuolar-type ATPases ( VMA5 , VMA9 and VMA11 ), vacuolar lipase ( ATG15 ) and α-mannosidase ( AMS1 ) were also upregulated ( Supplementary Table S7 ), which suggested that the cells initiated the turnover and recycling of intracellular components. The downregulated genes were related to primary metabolism, macromolecule metabolism and cellular metabolism, especially nucleobase, nucleoside, nucleotide and nucleic acid metabolic processes (GO: 0006139) and ribonucleoprotein complex biogenesis (GO: 0022613). Ribosome biogenesis is responsive to nutrient starvation through an evolutionarily conserved TOR signalling mechanism [31] , and for the 65 genes that were sampled by DGE and coded cytoplasmic ribosomal proteins, 39 genes were downregulated ( Fig. 3d , blue), which suggested that inhibition of the TOR complex suppressed the transcription of ribosomal components. Together, nitrogen limitation triggered a set of rescue pathways that included the induction of nitrogenous compound uptake, nitrogen assimilation, alternative nitrogen-source utilization, vacuolar protein degradation and autophagy, and inhibition of nitrogenous macromolecule biosynthesis. 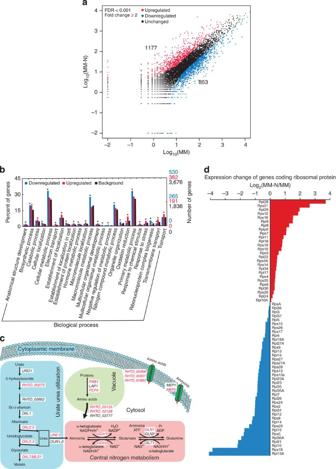Figure 3: Differential transcriptome ofR. toruloidesin response to nitrogen limitation. (a) Global profiling of gene expression changes. (b) Gene ontology enrichment analysis of differentially expressed genes. GO terms of biological process (level 3) were analysed and significantly enriched catalogues (when compared with the entire proteome, andP-value <0.05, Pearson'sχ2- test) are indicated with asterisks. (c) Expression changes (upregulation in red) of NCR-related genes. Pathways of urate and urea utilization, central nitrogen metabolism, vacuolar protein degradation and nitrogenous compound uptake were induced. (d) Relative expression levels (upregulation in red and downregulation in blue) of 65 ribosomal protein-encoding genes. Figure 3: Differential transcriptome of R. toruloides in response to nitrogen limitation. ( a ) Global profiling of gene expression changes. ( b ) Gene ontology enrichment analysis of differentially expressed genes. GO terms of biological process (level 3) were analysed and significantly enriched catalogues (when compared with the entire proteome, and P -value <0.05, Pearson's χ 2 - test) are indicated with asterisks. ( c ) Expression changes (upregulation in red) of NCR-related genes. Pathways of urate and urea utilization, central nitrogen metabolism, vacuolar protein degradation and nitrogenous compound uptake were induced. ( d ) Relative expression levels (upregulation in red and downregulation in blue) of 65 ribosomal protein-encoding genes. Full size image The regulation of central metabolism and lipid metabolism at the transcriptional level was also investigated ( Fig. 1 ; Supplementary Table S8 ). FAS in the MM-N sample was upregulated by 4.7- and 1.8-fold for FAS1 and FAS2 , respectively, but there were no significant differences in the expression of genes that were involved in the late stage of TAG biosynthesis. Isoprenoids are a variety of compounds (for example, steroids, carotenoids and terpenes) that are derived from the common precursor dimethylallyl diphosphate and its isomer 3-isopentenyl diphosphate. Four genes that are involved in isoprenoid backbone synthesis were upregulated in the MM-N sample ( Fig. 1 ). Indeed, the pink colour development of the culture was an indication of carotenoid biosynthesis. As lipids are highly reduced compounds, the supplement of a reducing power, mainly NADPH, is equally important to that of the precursor acetyl-CoA [6] . Activities of glucose-6-phosphate dehydrogenase ( ZWF1 ), 6-phosphogluconate dehydrogenase ( GND1 ), NADP + -dependent isocitrate dehydrogenase ( IDP1 ) and ME ( ME1 ) can generate NADPH. Although ZWF1 and IDP1 were upregulated by 1.9- and 4.8-fold, respectively, the expression of GND1 and ME1 were downregulated by 6.8- and 4.5-fold, respectively. The reduced transcriptional level of ME1 was consistent with early observations that indicated the expression of ME was suppressed during nitrogen exhaustion [32] , [33] . Interestingly, the expression of some genes that were involved in lipid degradation (that is, lipolysis, the β-oxidation cycle, and glyoxylate shunt) were also upregulated ( Fig. 1 ), which might be caused by free fatty acids being released by an elevated autophagy process [34] . We also compared the highly expressed genes of cells that were cultured in yeast-extract peptone dextrose (YPD), MM or MM-N media ( Fig. 4 ; Supplementary Table S10 ). It was found that the numbers of highly expressed genes were similar, and approximately half of those genes were shared by the three samples ( Fig. 4b , group G). The shared genes included those coding ribosomal proteins, actin, ACP ( RHTO_01048 ), TAL1 of the phosphopentose pathway, MDH1 and IDH2 of the tricarboxylic acid (TCA) cycle and GAPDH , ENO1 and FBA1 of glycolysis. Forty-two genes were highly expressed exclusively in the MM-N sample (group C) and included those encoding FAS1& 2 , PYC1 , GDH1 and acyl-CoA-binding protein ( RHTO_03853 ). Genes coding ACL1 and pyruvate dehydrogenase components ( LAT1 and LPD1 ) were highly expressed in the MM and MM-N samples (group E), where lipid contents were greater than 20%. 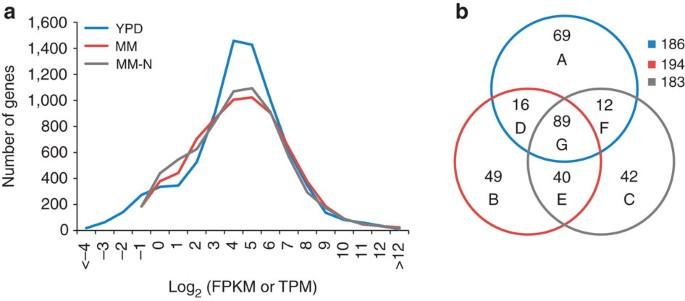Figure 4: Gene expression levels ofR. toruloidescultured in different media. (a) The histogram of gene expression levels that were normalized by FPKM for RNA-seq analysis (YPD) or by TPM for DGE analysis (MM and MM-N). (b) Venn diagram of highly expressed genes (FPKM or TPM >512) with specific numbers shown in groups A through G. Figure 4: Gene expression levels of R. toruloides cultured in different media. ( a ) The histogram of gene expression levels that were normalized by FPKM for RNA-seq analysis (YPD) or by TPM for DGE analysis (MM and MM-N). ( b ) Venn diagram of highly expressed genes (FPKM or TPM >512) with specific numbers shown in groups A through G. Full size image Comparative proteomic analysis In an earlier study, we performed comparative proteomic analysis of R. toruloides based on the proteome database of S. cerevisiae . As a result, 184 proteins were identified, and 46 of those proteins were found to change significantly during the lipid-production stage [35] . Here we re-analysed raw LC-MS/MS data that was based on the newly annotated protein data set that had been generated from the genomic data of R. toruloides . Although the previous analysis only cumulatively observed 184 proteins, in this study we observed 3,108 proteins, which amounted to roughly a 17-fold increment over the previous data set ( Supplementary Table S11 ). Thus, 38% of annotated genes were confirmed at the proteomic level. We were able to identify 2,057 proteins, which included over 32-fold more proteins than our previous data set ( Fig. 5a ; Supplementary Table S11 ). The intersection between the '24 h' and the '96 h' samples included approximately 100 more proteins than those of the other two intersections, which indicated that samples at the lipid-production stages more physiologically resembled each other. Further semi-quantitative analysis revealed 538 proteins that significantly varied in abundance between any two samples ( Fig. 5b and Supplementary Data 1 ). A good correlation was observed between protein expression levels of the '24 h' and the '96 h' samples, which had a Pearson's correlation coefficient of 0.79 ( Fig. 5c ) and suggested that many proteins were constantly expressed during lipid accumulation under nitrogen-limited conditions. 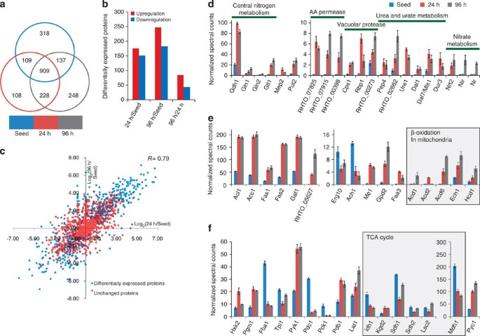Figure 5: Comparative proteomic analysis ofR. toruloidesduring lipid production. (a) The overlap of proteins (at least two occurrences within three replicates) that were identified by LC-MS/MS in the 'Seed' (the preculture, which was in YPD medium for 36 h; lipid content 9.8%), “24 h” (the culture in nitrogen-limited medium for 24 h; lipid content 37%) and '96 h' (the culture in nitrogen-limited medium for 96 h lipid content 63%) samples. (b) The number of differentially expressed proteins between the 'Seed', '24 h' and '96 h' samples. (c) Correlation analysis of proteins that were found in the '24 h' and '96 h' samples. (d) Upregulated proteins that were related to the NCR process. (e) Expression level changes of proteins that were involved in lipid metabolism. (f) Expression level changes of proteins that were involved in central carbon metabolism. The average±s.e.m. of the normalized spectral counts (y axis) is presented (ford,eandf). Figure 5: Comparative proteomic analysis of R. toruloides during lipid production. ( a ) The overlap of proteins (at least two occurrences within three replicates) that were identified by LC-MS/MS in the 'Seed' (the preculture, which was in YPD medium for 36 h; lipid content 9.8%), “24 h” (the culture in nitrogen-limited medium for 24 h; lipid content 37%) and '96 h' (the culture in nitrogen-limited medium for 96 h lipid content 63%) samples. ( b ) The number of differentially expressed proteins between the 'Seed', '24 h' and '96 h' samples. ( c ) Correlation analysis of proteins that were found in the '24 h' and '96 h' samples. ( d ) Upregulated proteins that were related to the NCR process. ( e ) Expression level changes of proteins that were involved in lipid metabolism. ( f ) Expression level changes of proteins that were involved in central carbon metabolism. The average±s.e.m. of the normalized spectral counts (y axis) is presented (for d , e and f ). Full size image Significantly higher levels were found for proteins linked to nitrogen metabolism under nitrogen-limited conditions. Specifically, proteins involved in nitrogenous compound transportation (Mep2, RHTO_07825, RHTO_07915, RHTO_00398, Dur3 and Nrt2), alternative nitrogen source utilization (proline, urate, urea and nitrate) and central nitrogen metabolism (Gdh1, Gln1, Gln2 and Glt1) were found at higher levels in the lipid-production samples than those in the 'Seed' sample ( Fig. 5d ), which suggested that nitrogen limitation alleviated the NCR process. On the other hand, the levels of ribosomal proteins, aminoacyl transfer RNA synthases, translation initiation and elongation factors, and protein folding-related proteins were reduced ( Supplementary Data 1 ), which indicated that the protein biosynthesis machinery was suppressed. The increased levels of vacuolar degradation- and autophagy-related proteins, such as vacuolar proteases (Cpb1, Rpb1 and Pep4), vacuolar-type ATPases (Vma2, Vma4, Vma13 and Stv1) and α-mannosidase (Ams1) suggested that an activated autophagy process was involved in responding to nitrogen starvation. The above-mentioned proteomic observations were also in good agreement with the differential transcriptomic data. Proteins involved in lipogenesis, especially for de novo fatty acid biosynthesis, were found at elevated levels ( Fig. 5e ). These proteins included Acl1, Me1, Acc1, Fas1 and Fas2 for fatty acid synthesis and glycerol-3-phosphate dehydrogenase isoform 2 (Gpd2) and glycerol-3-phosphate acyltransferase (Gat1) for glycerolipid synthesis. Cytosolic NADP + -dependent ME is the key enzyme that supplements NADPH for de novo lipogenesis [6] , [32] , [33] . Interestingly, although the transcription of ME1 was downregulated, the protein level of Me1 was significantly higher in the lipid production samples, which suggested that the regulation of ME activity was complicated. The level of acetyl-CoA synthase (Acs1) was increased by 2.2- and 2.1-fold in the '24 h' and '96 h' samples, respectively ( Fig. 6a ); however, levels of acetyl-CoA C-acetyltransferase (Erg10) and acetyl-CoA hydrolase (Ach1), which are the branch point enzymes for acetyl-CoA, were decreased. These data demonstrated that the acetyl-CoA flux was switched to the synthesis of fatty acids but not of isoprenoids. In fungi, a perilipin-like protein was characterized as a lipid-droplet protein that protected lipids from degradation [36] . RHTO_05627 was a perilipin family protein [37] that showed significantly higher levels at lipid-production stages, and the levels of proteins that were related to MBO were also increased, which was consistent with the upregulation of β-oxidation at the transcription level. 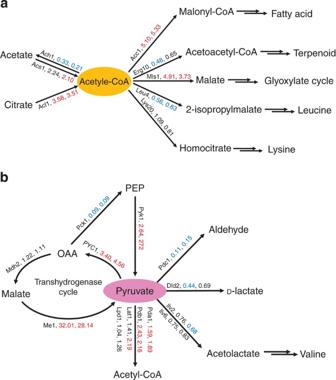Figure 6: Expression of acetyl-CoA- and pyruvate-associate enzymes. Fold changes in protein expression for enzymes at the branch points of acetyl-CoA (a) and pyruvate (b). Values represent the expression abundance ratios of '24h per Seed' and '96 h per Seed', respectively. Expression abundance ratios of significantly altered proteins (P-value <0.05,n=3, two-tailed, Student'st-test) are highlighted in red (increase) or blue (decrease). Figure 6: Expression of acetyl-CoA- and pyruvate-associate enzymes. Fold changes in protein expression for enzymes at the branch points of acetyl-CoA ( a ) and pyruvate ( b ). Values represent the expression abundance ratios of '24h per Seed' and '96 h per Seed', respectively. Expression abundance ratios of significantly altered proteins ( P -value <0.05, n =3, two-tailed, Student's t -test) are highlighted in red (increase) or blue (decrease). Full size image The levels of proteins associated with the TCA cycle (that is, Idh1, Sdh1, Sdh2 and Mdh1) decreased in the lipid-production samples ( Fig. 5f ), which was in agreement with early biochemical observations [6] , and the levels of proteins involved in pyruvate metabolism were significantly altered ( Figs 5f and 6b ). In the lipid-production samples, higher levels of pyruvate kinase (Pyk1) and pyruvate dehydrogenase components (Pdb1 and Lpd1) were found, whereas a lower level of pyruvate decarboxylase (Pdc1) was observed, which suggested that pyruvate was channelled to acetyl-CoA. Pyruvate carboxylase (PYC) functions as a key enzyme for the anaplerosis of the TCA cycle and gluconeogenesis. PYC was also proposed to be an essential part of the transhydrogenation machinery, which is composed of PYC, ME and malate dehydrogenase for the conversion of NADH to NADPH [6] . As the level of phosphoenolpyruvate carboxykinase (Pck1) that is responsible for the transformation of pyruvate to phosphoenolpyruvate was reduced, an increased level of Pyc1 should be mainly related to the NADPH supply for lipogenesis ( Fig. 6b ). Interestingly, enzymes catalysing these irreversible reactions in glycolysis (Hxk2 and Pyk1) were elevated. Moreover, the key enzyme in glycolysis, phosphofructokinase (Pfk1), was also augmented by 1.4-fold ( P -value <0.006, n =3 two-tailed, Student's t -test) at '24 h' and by 1.3-fold ( P -value <0.19, n =3 two-tailed, Student's t -test) at '96 h'. This evidence suggested that the glycolysis pathway would be slightly upregulated at lipid-production stages. Long-chain fatty acid derivatives have significant promise as drop-in biofuels and chemicals as replacements for petroleum products. In this regard, natural microbial hosts that produce neutral lipids such as TAGs should be explored, and the engineering of model microorganisms should be studied. The robustness of lipid production by the basidiomycetous fungus R. toruloides has been well-documented [10] , [14] , [38] . Auxotrophic mutants were achieved by physical and chemical mutagenesis [39] , and efficient transformation of R. toruloides with artificial plasmids has been demonstrated [40] . The current study disclosed the genome of R. toruloides based on deep sequencing and RNA-seq-assisted annotation, and further transcriptomic and proteomic analyses provided integrated information to discuss, for the first time and in much more detail, the molecular mechanism of fungi oleaginicity, nitrogen metabolism and the relationship between these processes. Some features of the R. toruloides genome that were linked to oleaginicity included the presence of ACL, split FAS, the perilipin family protein, and the MBO and carotenoid biosynthetic pathways. In R. toruloides , the expression level of ACL1 was extremely high ( Supplementary Table S8 ), which led to elevated citrate lysis activity for acetyl-CoA production. ACL 1 is an essential gene for oleaginicity and is absent in some Saccharomycetes fungi. Y. lipolytica , which is the only known species of the Saccharomyces that contains ACL, is an oleaginous yeast [41] . The presence of split FAS with two ACPs seemed conserved among oleaginous red yeasts ( Supplementary Fig. S10 ). Tandem ACPs were distributed broadly in polyketide synthases, and it was demonstrated that the yield of polyunsaturated fatty acids were dependent on the number of ACP domains [42] . Although it was unclear whether tandem ACPs in FAS would improve fatty acid production, this novel domain composition was to the best of our knowledge, first identified in FAS. Neutral lipids are stored in lipid droplets, which are specialized organelles that are coated with a phospholipid monolayer and proteins. Perilipin, a diverse family of lipid-droplet coating proteins, governs lipolysis [37] . In fungi, a perilipin-like protein MPL1 was characterized as a lipid-droplet protein that protected lipids from degradation [36] . The MPL1-like perilipins were exclusively found in pezizomycotinal ascomycetes such as Y. lipolytica , and the open-reading frame YALI0F24167g.aa (perilipin family protein, E-value 1.7e−05) of Y. lipolytica was identified in the most abundant fraction of the lipid-droplet proteome [43] . We found a new class of perilipin proteins, which was composed of the amino terminal perilipin and carboxy terminal apolipoprotein domains, in basidiomycetes ( Supplementary Fig. S11 ). During lipid accumulation, the expression of perilipin was consistent with the lipid amount and lipid-droplet volume ( Fig. 5e ), which suggested its importance to lipid accumulation. Nitrogen limitation has been extensively practiced to initiate lipid overproduction for oleaginous species [6] , [10] . Nitrogen limitation leads to amino acid (especially glutamine and leucine) starvation in the cytosol, which inhibits the activity of the TOR complex 1, a global regulator of nutrient signalling, by the Npr2/3 (ref. 31 ) or Gtr1/2 complexes (orthologues of the Rag protein) [44] . The conserved TOR complexes were present in R. toruloides ( Fig. 7a ) and the expression of NPR2 was indeed downregulated in this organism on nitrogen starvation ( Supplementary Table S7 ). Inactivated TORC1 then inhibits translation initiation and ribosome biogenesis and activates autophagy ( Fig. 7b ). As a result, protein synthesis is blocked and autophagy-related proteolysis is activated, which recycles amino acids. In S. cerevisiae , NCR-related genes are regulated by TOR signalling in response to nitrogen starvation through controlling the translocation of GATA transcription factors [45] . In the basidiomycetous fungus Cryptococcus neoformans , the GATA-type transcription factor Gat1 was also found to be responsible for nitrogen regulation [46] . Eleven putative GATA-type transcription factors were found in R. toruloides , and the HGATAR (H=A, C or T, and R=A or G) motif, which is recognized by GATA factors, was overrepresented in the upstream regions of those upregulated nitrogen metabolic genes ( Supplementary Fig. S12 ). Therefore, it would be interesting to characterize the roles of GATA factors in the transcriptional regulation of nitrogen metabolism in R. toruloides . Ribosome biogenesis and protein translation, the read-outs of TOR signalling, were also inhibited ( Fig. 3d and Supplementary Data 1 ); thus, nitrogen starvation resulted in blocked biosynthesis of nitrogenous macromolecules (that is, nucleic acids and protein). Inhibited TOR signalling cascades can also activate autophagy [29] , and a number of autophagy-related genes were induced on nitrogen starvation. As a result, free amino acids and fatty acids were expected to be released on degradation of proteins and membrane lipids, respectively. The free fatty acids might contribute to the activation of the MBO pathway for alternative acetyl-CoA production, and the free amino acids could contribute to relieving nitrogen stress. At the same time, autophagy was also demonstrated to have roles in lipid-droplet biogenesis [47] by making more room for lipid-droplet formation through the clearance of organelles or portions thereof ( Supplementary Fig. S6d,g ). 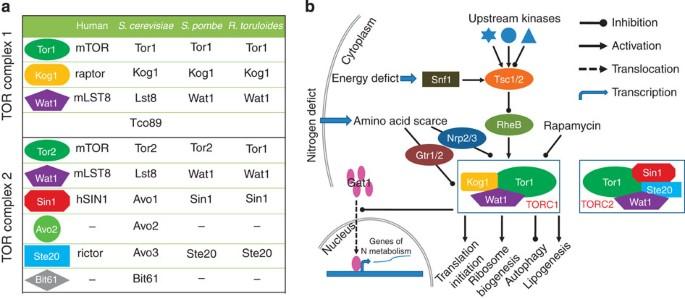Figure 7: TOR signalling links nitrogen regulation and lipid accumulation. (a) The components of TOR complexes. The TOR complexes ofR. toruloidesare similar to those ofSchizosaccharomyces pombeand mammals, but are different from those ofS. cerevisiae. (b) The proposed regulation model of lipid accumulation under nitrogen-limited conditions. Figure 7: TOR signalling links nitrogen regulation and lipid accumulation. ( a ) The components of TOR complexes. The TOR complexes of R. toruloides are similar to those of Schizosaccharomyces pombe and mammals, but are different from those of S. cerevisiae . ( b ) The proposed regulation model of lipid accumulation under nitrogen-limited conditions. Full size image Except for the upregulated transcription of FAS1 , FAS2 and PYC1 , under nitrogen-limiting conditions, some key genes for lipogenesis, such as ACL1 , ACC1 , ME1 , IDH1 and IDH2 , were not transcriptionally regulated, which was consistent with the transcriptomic analyses of the oleaginous yeast Y. lipolytica [19] . Comparative proteomic analysis would suggest that the regulation of these genes was post-transcriptional. We also found that cells at the lipid-production stage had elevated lipid-droplet wrapping, intensified glycolysis, an impaired TCA cycle and enhanced metabolic fluxes at branch points where pyruvate and acetyl-CoA were channelled into fatty acid biosynthesis. In addition, regulation of nitrogen metabolism at the transcriptional and proteomic levels included the following: (1) upregulation of genes involved in assimilation and transport of nitrogenous sources and genes for degradation/recycling of proteins or nitrogenous compounds, and (2) decreases in the biosynthesis of proteins and macromolecules. Although major evidence was found in the current study that support the classical opinion on nitrogen-limitation-mediated lipid production [6] , [23] , we now have a significantly broader and clearer view of microbial oleaginicity. This multi-omic information should aid the scientific community in genetic manipulation and metabolic engineering of lipid producers for the production of fatty acid derivatives that include tailor-made lipids, advanced fuel molecules [46] , microdiesel [5] and hydrocarbons [5] , [49] . Strain background The parent of the sequenced haploid strain R. toruloides NP11 was Y4 (ref. 10 ) and was derived from R. toruloides CGMCC 2.1389, which is identical to CBS 6016. Haploid NP11 ( MAT A1 ) and NP5-2 ( MAT A2 ) were isolated from basidiospores that were germinated from teliospores of Y4 ( Supplementary Fig. S13 ). Cell culture conditions and DNA/RNA sample preparation For genomic DNA preparation, R. toruloides was cultivated in YPD liquid medium (10 g l −1 yeast extract, 20 g l −1 peptone and 20 g l −1 dextrose) at 30 °C. Genomic DNA isolation was performed by following a previous protocol [50] . For cell disruption, the culture pellets were ground in liquid nitrogen or digested with MAN5C [51] followed by SDS and protease K (Takara) treatment. DNA was extracted by phenol (pH 8.0) and chloroform:isoamyl alcohol (24:1) and precipitated by ethanol (75%, v/v). The DNA samples were then dissolved in TE buffer (10 mM Tris–Cl, 1 mM EDTA, pH 7.6), incubated in the presence of RNase A (DNase-free, 20 μg ml −1 , Genview) at 37 °C for 30 min and extracted again. High-quality DNA (optical density (OD) 260/280 =1.8~2.0) that did not smear during electrophoresis was obtained, and the samples were lyophilized and delivered for genome sequencing. For massively parallel cDNA sequencing (RNA-seq), a chemostat culture of R. toruloides was run in a 3-l stirred tank reactor (Baoxing Bio-Engineering Equipment, Shanghai, China) that was equipped with an Inpro 6800 O 2 sensor and 405-DPAS-SC-K8S/225 pH electrode (Mettler Toledo). The cells were grown in YPD medium at 30 °C, pH 5.6, the airflow was 100 l h −1 (approximately 1 VVM) and the stirrer speed was 600 r.p.m., which maintained the dissolved oxygen at up to 70% of air saturation. The dilution rate was set at 0.5 h −1 , the feeding rate was maintained at 0.83 l h −1 and the working volume was 1.55 l, which made the growth rate similar to exponential growth in a shaking flask and resulted in a generation time of 2 h. Steady-state samples (OD 600 nm ~1.7) were harvested by centrifugation (6,200 g at 4 °C for 5 min) and cell pellets were frozen in liquid nitrogen. Total RNA was isolated using Trizol (Invitrogen) after grinding and was then treated with DNase I (RNase-free, NEB) to remove residual DNA [52] . The quality of the RNA was checked using an Agilent 2100 bioanalyser. For the 3′-tag DGE profiling, chemostat cultures of R. toruloides that were grown in minimal media were performed as aforementioned. The minimal medium (MM) was composed of 25 g l −1 glucose, 0.5 g l −1 MgSO 4 ·7H 2 O, 3 g l −1 KH 2 PO 4 and 5 g l −1 (NH 4 ) 2 SO 4 , whereas the nitrogen-limited medium (MM-N) contained the same components of the MM medium, but contained only 0.2 g l −1 (NH 4 ) 2 SO 4 as a nitrogen source and 6.3 g l −1 K 2 SO 4 to supplement the equivalent sulphur element. The culture conditions were set at 30 °C and pH 5.6, which was adjusted with 2 M KOH and 2% H 2 SO 4 . The dissolved oxygen was kept above 85% of air saturation, the stirrer speed was 500 r.p.m. and the airflow was 100 l h −1 . The dilution rate was 0.085 h −1 , which was much lower than that of the YPD culture. Sample harvesting and total RNA isolation were the same as that performed for RNA-seq, and the residual glucose and ammonium in the culture supernatants, dry cell weight and lipid content were measured as described previously [10] . Genome sequencing and assembly Four R. toruloides genomic DNA libraries with insert sizes of 200 bp, and 2 and 6 kb ( Supplementary Table S1 ) were constructed and sequenced in four lanes using the Illumina GAII or GAIIx sequencing platforms at BGI-Shenzhen. Approximately 5 Gb of data were obtained and assembled using the SOAPdenovo software [53] to generate 94 scaffolds that consisted of a total length of 20.2 Mb, close to the genome size of Rhodotorula graminis or Sporobolomycetes roseus ( Supplementary Fig. S14 ). The GenomeWalker Universal kit (Clontech) was used for genome walking to close the gaps between the scaffolds, and 34 scaffolds were obtained. Reads were aligned to the genome assembly using the Bowtie software [22] to estimate the sequencing depth. The CEGMA pipeline [21] was used to identify core eukaryotic genes. Massively parallel cDNA sequencing Initially, 10 μg of RNA was used to prepare the sequencing library using the Illumina mRNA-Seq 8-Sample Prep Kit (Illumina). The paired-end cDNA library with an insert length of 200±20 bp was sequenced using the Illumina HiSeq2000, and a total of 6.7 M paired-end reads of 90/90 bp in length were obtained ( Supplementary Table S1 ). RNA-seq reads were de novo assembled using SOAPdenovo (v1.04), and 78,979 contigs and 14,830 unigenes (≥200 bp), which were scaffolded and closed with paired-end reads, were obtained and re-aligned to the genomic sequence by BLAT [54] . A majority (98.6%) of the 17,814 assembled contigs (≥200 bp) could be mapped to the genome with more than 95% identity and 90% coverage. The raw reads were also mapped to the genome sequence using TopHat [55] and assembled ab initio using Cufflinks (v1.0.1) [56] . Genome annotation Initial gene prediction was done as described ( Supplementary Methods ). The first round of predictions and alignments were combined using GLEAN [57] to generate a consensus gene set with 6,469 gene models. An extra training using the GlimmerHMM and SNAP software was carried out to achieve sensitivity of ~90% and accuracy of ~60%, and were assessed with 269 independently annotated genes that were derived from the RNA-seq assembly. The gene predictions were also implemented using the Augustus software with the assistance of RNA-seq ( http://augustus.gobics.de/binaries/readme.rnaseq.html ), and all data were visualized and manually curated using the Argo software ( http://www.broadinstitute.org/annotation/argo/ ). The final set of genes was selected mainly on the basis of expression and homology ( Supplementary Fig. S4 ). For those genes that were merely predicted ab initio , consensus models from at least two predictions were reserved. The 3′- and/or 5′-untranslated regions were annotated if expressed, and finally 8,171 gene models were obtained. For gene expression analysis, the Cufflinks pipeline was used to estimate gene expression abundance and identify transcript isoforms when using option '-g'. Furthermore, the expression levels of genes and transcripts were normalized to FPKM (Fragments Per Kilobase of exon model per Million mapped fragments). Genes with alternatively spliced transcripts (1,371 were found) were also identified in silico . For gene function annotation, every predicted gene was annotated using the BLAST search engine against the non-redundant protein database at NCBI, the UniProtKB/Swiss-Prot database, the UniProtKB/Trembl database ( http://www.uniprot.org/ ) and KEGG genes database ( http://www.genome.jp/kegg/genes.html ). The domain and family of each protein was annotated via searching the InterPro database at EBI using InterProScan ( http://www.ebi.ac.uk/Tools/pfa/iprscan/ ), and Gene Ontology annotations were assigned using Blast2GO ( http://www.blast2go.com/b2ghome ). Gene function was classified by the eukaryotic orthologous group (KOG, http://www.ncbi.nlm.nih.gov/COG/ ), and the automatic assignment of metabolic pathway was implemented by KAAS ( http://www.genome.jp/tools/kaas/ ). 3′-Tag DGE profiling The Nla III libraries were prepared using the Illumina Tag Profiling Sample Prep Kits (Illumina) and were sequenced on the Illumina GAIIx platform with read lengths of 35 bp. More than three million reads were obtained ( Supplementary Table S1 ) and analysed in silico using the in-house Perl pipeline that was developed by BGI-Shenzhen. In brief, a database with all sense and antisense tags (CATG+17 nucleotides) of the annotated transcripts was created. The raw reads were processed to filter out low-quality tags and adaptor sequences, and subsequently, clean tags that contained CATG and an additional 17 bp were counted and mapped to the tag database of transcriptomic or genomic sequences without more than 1 bp mismatch. For transcript quantification, tags that occurred only once or had multiple hits to transcripts were discarded, and tags that mapped to the same transcript regardless of their positions were counted and normalized to tags per million (TPM). To identify differentially expressed genes, the rigorous algorithm Audic and Claverie's [58] test, which was described previously, was used to test for significance. In addition, the false discovery rate (FDR) adjustment was used to control the error rate, a threshold of 0.001 for FDR and a fold change of 2 was set as the criteria for differentially expressed genes. We found 1,177 and 853 genes that were upregulated and downregulated, respectively. Proteomic analysis Proteomic data from a previous study were analysed using the newly annotated protein data set [35] . MS/MS spectra data were searched against the protein database of R. toruloides using SEQUEST as described [35] . The results were filtered using the SFOER software with optimized criteria [59] , and the corresponding FDR was below 1%. In total, 3,108 proteins were identified using at least one peptide, and 2,057 proteins that occurred more than twice in the triplicate analyses were counted as expressed proteins. For semi-quantitative comparison, the spectral counts of proteins that were identified in all three replications were used and normalized, and combined statistical tests were applied to assess the significance [60] . Proteins with a fold change >2, a P -value <0.05 for the t -test and a G -value >1.35 for the G-test (corresponding to 3.9 for raw spectral counts) of each of the two samples were assigned as differentially expressed proteins, and this analysis led to 538 proteins that showed significant level changes. Accession codes : This Whole Genome Shotgun Sequencing project has been deposited into DDBJ/EMBL/GenBank under the accession number ALAU00000000 . The version that is described in this paper is the first version, ALAU01000000. Raw reads of the WGS sequencing and RNA-seq analysis have been deposited into the NCBI Sequence Read Archive (SRX156633–SRX156637). DGE profiling data have been deposited into NCBI's Gene Expression Omnibus and was given the accession number GSE39023 . The proteomic data that is associated with this manuscript may be downloaded from ProteomeCommons.org Tranche using the following hash: HzAX+3G+zoH9LngqJ+29NyszSltcjGUyxKWjNhCIRKOab/G0LG9Kw15quSpAteJOio7+ V2tR9O3vt9pyHyu1O9/I54gAAAAAAAA43A==. All data are also available at http://www.bioconversion.dicp.ac.cn/EWEB/ZZW-data.html . How to cite this article: Zhu, Z et al . A multi-omic map of the lipid-producing yeast Rhodosporidium toruloides . Nat. Commun. 3:1112 doi: 10.1038/ncomms2112 (2012).